Select interneuron clusters determine female sexual receptivity inDrosophila Female Drosophila with the spinster mutation repel courting males and rarely mate. Here we show that the non-copulating phenotype can be recapitulated by the elimination of spinster functions from either spin-A or spin-D neuronal clusters, in the otherwise wild-type ( spinster heterozygous) female brain. Spin-D corresponds to the olfactory projection neurons with dendrites in the antennal lobe VA1v glomerulus that is fruitless -positive, sexually dimorphic and responsive to fly odour. Spin-A is a novel local neuron cluster in the suboesophageal ganglion, which is known to process contact chemical pheromone information and copulation-related signals. A slight reduction in spinster expression to a level with a minimal effect is sufficient to shut off female sexual receptivity if the dominant-negative mechanistic target of rapamycin is simultaneously expressed, although the latter manipulation alone has only a marginal effect. We propose that spin-mediated mechanistic target of rapamycin signal transduction in these neurons is essential for females to accept the courting male. Female partner preference is believed to be a major driving force for the creation of male-specific morphology and behaviour that improve the reproductive success of males [1] . One of the factors modulating female partner preference is sexual receptivity, the physiological mechanism of which has been poorly understood. Except for a few days after eclosion, wild-type virgin females in Drosophila melanogaster copulate when courted by a male [2] . In contrast, females with the spinster (spin) mutation resist copulating. The spin mutant females display a variety of rejection behaviours against a courting male, such as decamping, fending with the legs, flicking of the wings, kicking, curling the abdomen and spreading the vaginal plate [3] , [4] . In this study, we intend to identify the central nervous system neurons that control sexual receptivity and thus partner preference of female flies by producing a small number of spin mutant homozygous cells in the otherwise spin heterozygous brain, with the expectation that such spin -mosaic virgin females that have spin mutant clones in the ‘receptivity centre’ will repel a courting male in contrast to the remainder mosaic females with spin mutant clones in the brain regions unrelated to receptivity. The unambiguous behavioural phenotype is a prerequisite for this type of analysis and spin mutants suffice this requirement. To generate spin mutant clones we adopted mosaic analysis with a repressible cell marker (MARCM) [5] , with which the decision-making centre for male courtship behaviour has been identified [6] , [7] . Our analysis successfully identify two interneuron groups that induce non-copulating phenotype in females when they are homozygous for the spin mutation. We identify the spin-D group, which is composed of second-order olfactory projection neurons that relay the conspecific odour information, and the spin-A group, which represents a local neuron cluster confined in the suboesophageal ganglion. We propose that spin functions as a molecular switch in these neurons to convert the female physiology from the sexually non-receptive to receptive state and to coordinate the associated changes in mating behaviour. Neural and glial Spin coordinately regulates receptivity The receptivity of spin mutant females is restored by spin + overexpression, as driven by spin-GAL4 with expression in both glia and neurons ( Fig. 1a–c ). To determine whether the expression in glia or neurons or both is crucial for the spin behavioural role, we attempted to rescue the mutant phenotype by selectively overexpressing spin + in neurons with elav c155 (referred to as elav-GAL4 hereafter) or in glia with repo-GAL4 . The results indicated that neuronal but not glial overexpression of spin + restores the receptivity that has been reduced by the spin mutation ( Fig. 1d ). In the second set of experiments, spin functions were knocked down in either neurons or glia by forcibly expressing UAS-spin RNAi as driven by elav-GAL4 or repo-GAL4 . The flies were raised at 29 °C to enhance transgene expression and tested for mating behaviour at 25 °C. We found that the spin RNAi expressed in neurons but not that expressed in glia attenuated the sexual receptivity of wild-type females ( Fig. 1e ). To further evaluate the possible involvement of spin function in glia, spin was knocked down in both neurons and glia in flies raised at 25 °C, a temperature expected to result in low-level expression of transgenes. Interestingly, when spin RNAi was expressed in both neurons and glia, female sexual receptivity dramatically declined even in these female flies raised at 25 °C ( Fig. 1f ), the temperature at which no effect was detected if spin RNAi was targeted to either neurons or glia. We conclude that female receptivity is established by spin functions primarily in neurons while glial spin has a subsidiary role. 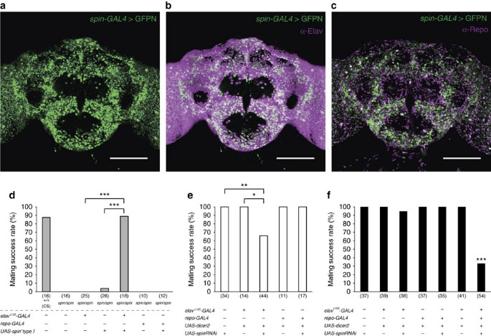Figure 1: Contributions of neuronal and glial Spin to female sexual receptivity. (a)spin-GAL4expression in the adult female brain was detected with nuclear-targeted GFP (GFPN). (b,c)spin-GAL4-expressing cells are composed of anti-Elav-positive neurons (magenta inb) and anti-Repo-positive glia (magenta inc) in the adult female brain. (d) The effectiveness ofUAS-spin+type Iin rescuing the non-copulating phenotype ofspinP1mutant females was estimated by expressing it in neurons withelavc155or in glia withrepo-GAL4. Wild-type (CS, Canton-S) and other control flies were also examined. Thespingene produces five isoforms, Spin I—V, only two of which (Spin I and Spin V) have been demonstrated to rescue the sexual receptivity phenotype4. Transgenes the fly carried are shown at the bottom; + and — indicate the presence and absence of the indicated transgene in each fly group. The number of flies examined is shown in parentheses. The female sexual receptivity was measured by the percentage of pairs copulating within a 1-h observation period at 25 °C. (e) The effect ofspinknockdown in either neurons or glia on sexual receptivity when the flies were raised at 29 °C to attain higher levels of transgene expression. Dicer2 was also used to enhance the RNAi effect. Neuronal but not glial expression of RNAi was effective in reducing sexual receptivity. (f) When the flies were raised at 25 °C, transgene expression levels would be lower than at 29 °C,spinRNAi expression in either neurons or glia had no discernible effect on receptivity, while its simultaneous expression in both neurons and glia reduced sexual receptivity. The statistical significance of differences was evaluated by the Fisher’s exact probability test with Bonferroni correction (***P<0.001; **P<0.01; *P<0.05). Simultaneousspinknockdown in neurons and glia was not possible at 29 °C because practically no adult flies were recovered for lethality. Scale bar, 100 μm fora–c. Figure 1: Contributions of neuronal and glial Spin to female sexual receptivity. ( a ) spin-GAL4 expression in the adult female brain was detected with nuclear-targeted GFP (GFPN). ( b , c ) spin-GAL4 -expressing cells are composed of anti-Elav-positive neurons (magenta in b ) and anti-Repo-positive glia (magenta in c ) in the adult female brain. ( d ) The effectiveness of UAS-spin + type I in rescuing the non-copulating phenotype of spin P1 mutant females was estimated by expressing it in neurons with elav c155 or in glia with repo-GAL4 . Wild-type (CS, Canton-S) and other control flies were also examined. The spin gene produces five isoforms, Spin I—V, only two of which (Spin I and Spin V) have been demonstrated to rescue the sexual receptivity phenotype [4] . Transgenes the fly carried are shown at the bottom; + and — indicate the presence and absence of the indicated transgene in each fly group. The number of flies examined is shown in parentheses. The female sexual receptivity was measured by the percentage of pairs copulating within a 1-h observation period at 25 °C. ( e ) The effect of spin knockdown in either neurons or glia on sexual receptivity when the flies were raised at 29 °C to attain higher levels of transgene expression. Dicer2 was also used to enhance the RNAi effect. Neuronal but not glial expression of RNAi was effective in reducing sexual receptivity. ( f ) When the flies were raised at 25 °C, transgene expression levels would be lower than at 29 °C, spin RNAi expression in either neurons or glia had no discernible effect on receptivity, while its simultaneous expression in both neurons and glia reduced sexual receptivity. The statistical significance of differences was evaluated by the Fisher’s exact probability test with Bonferroni correction (*** P <0.001; ** P <0.01; * P <0.05). Simultaneous spin knockdown in neurons and glia was not possible at 29 °C because practically no adult flies were recovered for lethality. Scale bar, 100 μm for a – c . Full size image Two neuronal clusters determine female sexual receptivity To determine which neurons are involved in making the female flies sexually receptive, we conducted MARCM [5] in which spin mutant clones were produced in the brain of spin heterozygous females, which were subjected to mating behaviour assays and subsequent histology to identify the neurons that were spin mutant clones ( Fig. 2 ). Among the 902 mosaic females subjected to mating assays, 7 flies did not copulate in a 1-h observation period and the remaining 895 flies copulated. In our experimental design, only cells mutant for spin were labelled with mCD8::GFP. These cells showed strong lysotracker staining ( Fig. 3 ), in keeping with the reported spin mutant phenotype [8] , [9] . Labelling the brains from these seven non-receptive females revealed several neuronal clusters that were mCD8::GFP positive in more than three flies, implying that some of these clusters are pivotal in regulating female receptivity; these included eight clusters that are reliably identifiable across different flies based on the location of their somata and neurite projections, and we named these clusters spin-A, -B, -C, -D, -E, -F, -G and -H, respectively ( Fig. 2a–f ). To assess whether any of these clusters indeed contributes to the determination of sexual receptivity levels, we compared the frequency of homozygous (mCD8::GFP positive) cells in the respective clusters between the copulating and non-copulating mosaic fly groups. If any of these clusters have a strong impact on the sexual receptivity levels, then one can anticipate that such a cluster will be spin homozygous (mCD8::GFP positive) at a significantly higher frequency in the non-copulating fly group than in the copulating fly group. It turned out that the frequency of spin mutant homozygosity was significantly higher in the spin-A and -D clusters of the non-copulating fly group than in those of the copulating fly group ( Fig. 2g ), but this relation was not observed for the other clusters. We have no evidence that some other clusters need to be spin mutant homozygous in addition to the spin-A and -D cluster in order to make the mosaic female unreceptive to a courting male ( Table 1 ). We conclude that the spin-A and -D clusters participate in the regulation of female sexual receptivity. 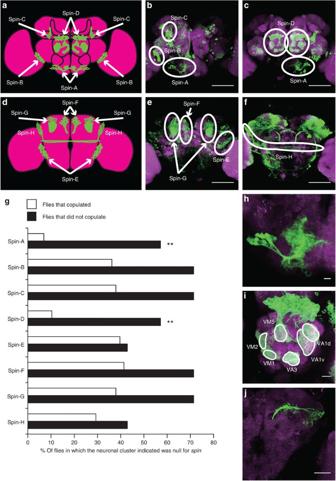Figure 2: Two neuronal clusters reduced receptivity when homozygous forspinin the otherwisespinheterozygous brain. (a–f) Eight neural clusters repeatedly labelled asspinmutant cells were present in non-copulating mosaic females. Four clusters (spin-A to -D) in the anterior brain shown as a schematic (a) or reconstructed images (b,c). Another four clusters (spin-E to -H) in the posterior brain shown as a schematic (d) or reconstructed images (e,f). Scale bar, 100 μm. (g) The proportions of flies in which the indicated clusters werespinhomozygous in the two fly groups, that is, copulating flies (open bars) and non-copulating flies (filled bars). Female flies that did not copulate within a 1-h observation period were classified as ‘non-copulating.’ By examining 902 mosaic females, we recovered seven non-copulating females that were then used to estimate thespin-homozygous ratio for each neuron cluster. To determine the neuronalspin-homozygous ratio for copulating flies, the brains from 58 flies were scored. These 58 flies were arbitrarily chosen from fly pools that yielded a non-copulating mosaic fly. Pairwise comparisons of thespinmutant ratio between the copulating and non-copulating groups for each cell cluster revealed statistically significant differences only in the spin-A and -D clusters. The statistical significance of differences was evaluated by the Fisher’s exact probability test (**P<0.01). (h) The structure of spin-A cluster neurons labelled as a MARCM clone. (i,j) The structure of spin-D cluster neurons labelled as a MARCM clone, which are shown for somata and dendrites in antennal lobe glomeruli (VA1d, VA1v, VA3, VM1, VM2 and VM5;i) and for axons projecting to the mushroom body and lateral horn (j). Scale bar, 10 μm (h,i) and 50 μm (j). Figure 2: Two neuronal clusters reduced receptivity when homozygous for spin in the otherwise spin heterozygous brain. ( a – f ) Eight neural clusters repeatedly labelled as spin mutant cells were present in non-copulating mosaic females. Four clusters (spin-A to -D) in the anterior brain shown as a schematic ( a ) or reconstructed images ( b , c ). Another four clusters (spin-E to -H) in the posterior brain shown as a schematic ( d ) or reconstructed images ( e , f ). Scale bar, 100 μm. ( g ) The proportions of flies in which the indicated clusters were spin homozygous in the two fly groups, that is, copulating flies (open bars) and non-copulating flies (filled bars). Female flies that did not copulate within a 1-h observation period were classified as ‘non-copulating.’ By examining 902 mosaic females, we recovered seven non-copulating females that were then used to estimate the spin -homozygous ratio for each neuron cluster. To determine the neuronal spin -homozygous ratio for copulating flies, the brains from 58 flies were scored. These 58 flies were arbitrarily chosen from fly pools that yielded a non-copulating mosaic fly. Pairwise comparisons of the spin mutant ratio between the copulating and non-copulating groups for each cell cluster revealed statistically significant differences only in the spin-A and -D clusters. The statistical significance of differences was evaluated by the Fisher’s exact probability test (** P <0.01). ( h ) The structure of spin-A cluster neurons labelled as a MARCM clone. ( i , j ) The structure of spin-D cluster neurons labelled as a MARCM clone, which are shown for somata and dendrites in antennal lobe glomeruli (VA1d, VA1v, VA3, VM1, VM2 and VM5; i ) and for axons projecting to the mushroom body and lateral horn ( j ). Scale bar, 10 μm ( h , i ) and 50 μm ( j ). 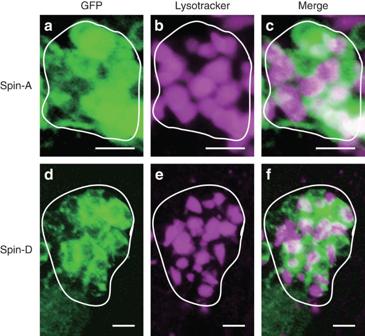Figure 3: Spin-A and -D MARCM clones examined for the expression of lysotracker. GFP fluorescence monitoringspin-GAL4expression (left-hand side panel), lysotracker signals (middle panel) and their merged image (right-hand side panel) are shown for spin-A (a–c) and spin-D (d–f) clusters that arespinmutant clones generated by MARCM. Scale bar, 5 μm. Full size image Figure 3: Spin-A and -D MARCM clones examined for the expression of lysotracker. GFP fluorescence monitoring spin-GAL4 expression (left-hand side panel), lysotracker signals (middle panel) and their merged image (right-hand side panel) are shown for spin-A ( a – c ) and spin-D ( d – f ) clusters that are spin mutant clones generated by MARCM. Scale bar, 5 μm. Full size image Table 1 Genotype combinations of spin-A to spin-H clusters in seven mosaic flies that did not copulate. Full size table Close inspection of the mCD8::GFP-labelled spin-D clones revealed that this cluster is composed of secondary projection neurons with dendritic fields in the antennal lobe ( Fig. 2i ) while extending their axons towards the lateral horn ( lh ) via the mushroom body ( Fig. 2j ). Single clones of the spin-D cluster from different mosaic flies share six glomeruli that are positive for mCD8::GFP, that is, VA1d, VA1v, VA3, VM1, VM2 and VM5 ( Fig. 2i ). As every projection neuron is known to innervate a single glomerulus [10] , the spin-D cluster is considered to be a composite of six distinct types of projection neurons. On the other hand, the spin-A cluster represents a hitherto undescribed group of some 35–45 local neurons confined to the suboesophageal ganglion ( Fig. 2h ). Labelling of the spin-A cluster was inhibited by Choline-acetyltransferase-GAL80 ( Chat-GAL80 ) ( Fig. 4a ) and thus the neurons composing this cluster are likely to be cholinergic. Arbours of the spin-A cluster neurons interdigitate with axon terminals of ppk -positive neurons ( Fig. 4c and Supplementary movie 1 ) whose origin remains obscure. 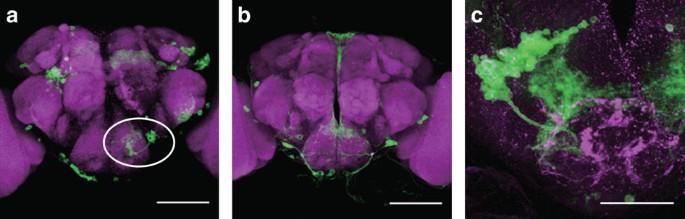Figure 4: Anatomical and neurochemical characteristics of spin-A cluster neurons. (a) The spin-A cluster was labelled with mCD8::GFP (circled). (b) The spin-A cluster was never labelled when the fly carriedChat-GAL80, which inhibits the GAL4 function in cholinergic neurons. Anterior view. Scale bar, 100 μm. (c) Spin-A cluster neurons have arborizations interdigitating withppk-positive axon terminals. Theppk-mCherryfusion gene was used to labelppkneurons in the brain that carried a spin-A MARCM clone marked with mCD8::GFP. Scale bar, 50 μm. Green:spin-GAL4-positive cells (a–c). Magenta: neuropil staining with nc82 (a,b) or mCherry expression (c). Figure 4: Anatomical and neurochemical characteristics of spin-A cluster neurons. ( a ) The spin-A cluster was labelled with mCD8::GFP (circled). ( b ) The spin-A cluster was never labelled when the fly carried Chat-GAL80 , which inhibits the GAL4 function in cholinergic neurons. Anterior view. Scale bar, 100 μm. ( c ) Spin-A cluster neurons have arborizations interdigitating with ppk -positive axon terminals. The ppk-mCherry fusion gene was used to label ppk neurons in the brain that carried a spin-A MARCM clone marked with mCD8::GFP. Scale bar, 50 μm. Green: spin-GAL4 -positive cells ( a – c ). Magenta: neuropil staining with nc82 ( a , b ) or mCherry expression ( c ). Full size image Or47b olfactory pathway regulates sexual receptivity We wanted to determine whether all six types of projection neurons in the spin-D cluster are involved in female sexual receptivity, or only a few of these types are important. As no tool is available to manipulate each type of projection neurons separately, we instead attempted to prevent select projection neurons from receiving normal synaptic inputs by expressing a neural activity blocker or spin RNAi in primary afferents, for which distinct Or-GAL4 s can be used to separately manipulate sensory inputs to different glomeruli. The six glomeruli involving the spin-D cluster have been known to receive inputs from the following sensory neurons, each of which expresses a specific Ors [11] , [12] : Or88a (VA1d), Or47b (VA1v), Or67b (VA3), unidentified (VM1), Or43b (VM2) and Or98a (VM5). We compared the effect of forced expression of an activated form of the inward rectifier K channel Kir2.1 ( [13] ), which hyperpolarizes the membrane and inhibits neural excitation, on female sexual receptivity when driven by five different Or-GAL4s, that is, Or88a-GAL4 (VA1d), Or47b-GAL4 (VA1v), Or67b-GAL4 (VA3), Or43b-GAL4 (VM2) and Or98a-GAL4 (VM5). The results showed that Or98a- or Or47b-neurons, when inhibited, significantly retarded the copulation initiation, whereas Or43b-, Or67b- and Or88a-neurons did not ( Fig. 5 ). The negative effect on the copulation success of inhibiting Or47b neurons was more pronounced compared with that of Or98a neurons ( Fig. 5b versus 5e ). Our preliminary findings show that rather unexpectedly, the reduced female receptivity caused by the inhibition of Or47b neurons was not further reduced by the additional inhibition of Or98a neurons (data not shown). 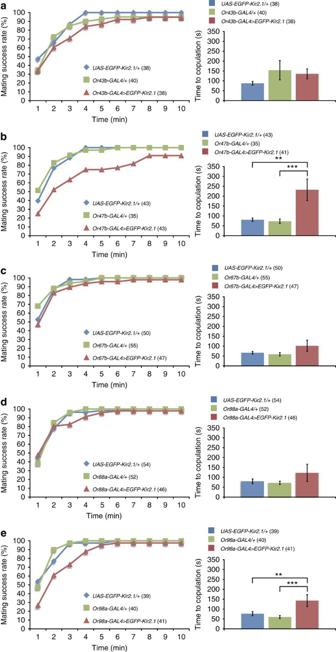Figure 5: Differential effects of blocking olfactory receptor neuronal activity on sexual receptivity. The cumulative number of pairs copulating over time (relative to the total pairs observed: left-hand side graphs) and the time to copulation (mean±s.e.m: right-hand side graph) were compared among the females in which olfactory receptor neurons expressing either Or43b (a), Or47b (b), Or67b (c), Or88a (d) or or98a (e) were prevented from firing. The statistical significance of differences was evaluated by the Kruskal–Wallis analysis of variance followed by Scheffe’s F test for the measure of time to copulation (***P<0.001; **P<0.01). The number of flies examined is shown in parentheses. Figure 5: Differential effects of blocking olfactory receptor neuronal activity on sexual receptivity. The cumulative number of pairs copulating over time (relative to the total pairs observed: left-hand side graphs) and the time to copulation (mean±s.e.m: right-hand side graph) were compared among the females in which olfactory receptor neurons expressing either Or43b ( a ), Or47b ( b ), Or67b ( c ), Or88a ( d ) or or98a ( e ) were prevented from firing. The statistical significance of differences was evaluated by the Kruskal–Wallis analysis of variance followed by Scheffe’s F test for the measure of time to copulation (*** P <0.001; ** P <0.01). The number of flies examined is shown in parentheses. Full size image We next examined the effect of knockdown of spin in Or98a-, Or47b-, Or43b-, Or67b- or Or88a-neurons on female sexual receptivity. In this series of experiments, repo-GAL4 was combined with each Or-GAL4 to drive spin RNAi expression, because simultaneous knockdown of spin in neurons and glia was most effective in reducing female sexual receptivity ( Fig. 6a–e ). As can be seen in Fig. 6a–e , Or47b neurons, but none of the other four olfactory receptor neurons, attenuated female sexual receptivity when spin knockdown was achieved ( Fig. 6a–e ). We conclude that the olfactory pathway mediated by the Or47b neurons and the projection neurons with dendrites in the VA1v glomerulus has a key role in determining the level of female sexual receptivity. Among the five Ors examined, Or47b and Or88a are the receptors known to respond to conspecific fly odour (other Ors are activated by food odour, for example) [14] , and VA1v is one of the three sexually dimorphic glomeruli [15] , [16] and expresses fruitless ( fru ) [16] , a major control gene for the courtship circuitry [17] , [18] . Notably, spin knockdown in Or47b neurons reduced but did not block female sexual receptivity, in contrast to the spin mutant females, in which no copulation was observed. This is presumably because the neural pathway involving spin-A cluster neurons remained functional even after the spin-D pathway was impaired by the spin knockdown in Or47b neurons, whereas in spin mutant females both the spin-A and -D pathways were disrupted. 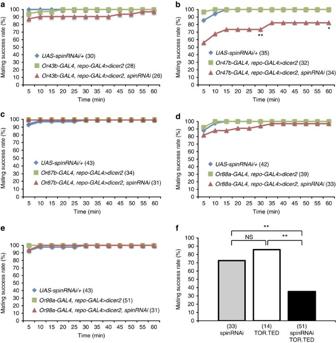Figure 6: The effect ofspinRNAi expressed in olfactory receptor neurons and of mTOR inhibition on sexual receptivity. (a–e) The cumulative number of pairs copulating over time (relative to the total pairs observed) was compared among the females in whichspinRNAi was expressed in olfactory receptor neurons expressing either Or43b (a), Or47b (b), Or67b (c), Or88a (d) or Or98a (e). Note thatrepo-GAL4andUAS-dicer2were used to enhance the effect ofspinRNAi on sexual receptivity. The statistical significance of differences was evaluated by the Fisher’s exact probability test with Bonferroni correction for the cumulative copulation success (**P<0.01; *P< 0.05). (f) Synergy ofmTorandspinin the regulation of female receptivity. Although the mating success rate in a 1-h observation period was only moderately reduced by theelav-GAL4-mediated expression of either dominant-negativemTor(TOR.TED, 85.7%;n=14) orspinRNAi (spinRNAi; 72.7%;n=33), simultaneous expression of these two (TOR.TED+spinRNAi) resulted in a marked decrease in the receptivity (35.3%;n=51). The statistical differences were evaluated by the Fisher’s exact probability test with Bonferroni correction, or by theχ2-test for the comparison in which the expectation frequency exceeded 5 in all parameters (**P<0.01; not significant (NS)P>0.05). The number of flies examined is shown in parentheses. Figure 6: The effect of spin RNAi expressed in olfactory receptor neurons and of mTOR inhibition on sexual receptivity. ( a – e ) The cumulative number of pairs copulating over time (relative to the total pairs observed) was compared among the females in which spin RNAi was expressed in olfactory receptor neurons expressing either Or43b ( a ), Or47b ( b ), Or67b ( c ), Or88a ( d ) or Or98a ( e ). Note that repo-GAL4 and UAS-dicer2 were used to enhance the effect of spin RNAi on sexual receptivity. The statistical significance of differences was evaluated by the Fisher’s exact probability test with Bonferroni correction for the cumulative copulation success (** P <0.01; * P < 0.05). ( f ) Synergy of mTor and spin in the regulation of female receptivity. Although the mating success rate in a 1-h observation period was only moderately reduced by the elav-GAL4 -mediated expression of either dominant-negative mTor (TOR.TED, 85.7%; n =14) or spin RNAi (spinRNAi; 72.7%; n =33), simultaneous expression of these two (TOR.TED+spinRNAi) resulted in a marked decrease in the receptivity (35.3%; n =51). The statistical differences were evaluated by the Fisher’s exact probability test with Bonferroni correction, or by the χ 2 -test for the comparison in which the expectation frequency exceeded 5 in all parameters (** P <0.01; not significant (NS) P >0.05). The number of flies examined is shown in parentheses. Full size image Mechanistic target of rapamycin signalling is required for normal sexual receptivity spin knockdown in Or47b neurons is much more effective in reducing sexual receptivity than neural activity block in the same group of neurons ( Fig. 5b versus Fig. 6b ). This implies that Spin signalling in the neurons is pivotal for regulating sexual receptivity. As Spin has been shown to activate mechanistic target of rapamycin (mTOR) in starvation-induced autophagy [19] , [20] , we examined the possible effect of mTor inactivation on spin -dependent sexual receptivity. When spin or mTor was singly knocked down, females exhibited only a moderate reduction in receptivity ( Fig. 6f ). In contrast, when both spin and mTor were knocked down simultaneously, the females showed a striking reduction in receptivity ( Fig. 6f ). This synergistic effect of spin and mTor supports the hypothesis that these two proteins cooperate to regulate female sexual receptivity. In this study, we identified two groups of neurons whose malfunction resulted in a significant decline in female sexual receptivity: a population of olfactory projection neurons with its dendritic field in the VA1v glomerulus of the antennal lobe (spin-D) and a cluster of local neurons in the suboesophageal ganglion (spin-A). It is of interest to note that the location of projection neuron somata appears to coincide with SP11, to which Tompkins and Hall [21] assigned the role of controlling female sexual receptivity by classical mosaic analysis. VA1v is one of the three fru -expressing sexually dimorphic glomeruli [15] , [16] and receives synapses from Or47b neurons that are known to respond to a conspecific odour common to both sexes [14] . It is therefore likely that the Or47b-VA1v sensory pathway participates in the species recognition rather than in the discrimination of the sex within the species. A recent study showed that wild-type males, but not Or47b mutant males, vigorously court a hydrocarbon-deficient target male and this courtship is suppressed when the target male has been perfumed with 7-tricosene (7-T) ( [22] ), a male-predominant pheromone, which is also present in females at a low level. This observation suggests the intriguing possibility that Or47b neurons accelerate mating in both females and males by responding to compounds common to both sexes, and that the excitatory state produced by Or47b neuron activities is modulated negatively by 7-T in males and positively by 7-T in females. In fact, 7-T has been shown to enhance female sexual receptivity, and amputation of the female antennae abrogates this effect of 7-T ( [23] ). On the other hand, Or47b neurons do not respond to a male-specific pheromone, cis -vaccenyl acetate [14] , which reportedly accelerates female acceptance of a courting male [24] . Or47b neurons make synapses in the VA1v glomerulus on the projection neurons extending axons to a region in the lh pheromone responsive field that is sexually dimorphic [10] . In this region, many fru -expressing neurons intersect and some of the command outputs to control courtship are likely initiated there, at least in males [7] , [25] , [26] . On the other hand, the local interneurons composing the spin-A cluster have not been described previously, and thus nothing is known about their input–output relationships. The suboesophageal ganglion is well-known as the centre for gustation, which has a central role in pheromone perception in mating [27] . Recent studies have suggested that, upon copulation, the ppk and fru double-positive uterine mechanosensory neurons projecting to the ventral ganglia trigger the conversion of female physiology and behaviour from the virgin type to the mated type [28] , [29] . In this study, we found that spin-A cluster neurons potentially receive inputs from ppk -positive neurons of a non-uterus origin ( Fig. 4c and Supplementary movie 1 ), whose roles in female receptivity need to be addressed. In addition, a few dsx -expressing interneurons in the ventral ganglia with an ascending axon that terminates in the suboesophageal ganglion have been implicated in the control of female sexual receptivity [30] . Therefore, it is envisaged that the spin-A cluster neurons integrate multiple sensory inputs for switching the female physiology and behaviour upon copulation and their outputs are relayed by the ascending interneurons to the brain. Spin-A cluster neurons express neither fru nor dsx , and, therefore, are unlikely to be sexually dimorphic. It is tempting to speculate that the spin-A cluster originally engaged in metabolic homoeostasis later became a key regulator of sexual receptivity, specifically in females, where this cluster had become integrated into a female-specific circuitry that controls mating behaviour. We found that the reduction in female sexual receptivity was much more pronounced when spin was knocked down than when neuronal activity was suppressed in Or47b neurons ( Figs 5b and 6b ). It might be that spin knockdown impaired neural development, leading to a more severe phenotype than that induced by the acute inhibition of neural activities. Note, however, that no apparent structural deficits were detected in spin -homozygous neurons that had developed as a MARCM clone in the otherwise heterozygous background, even though they exhibited high levels of lysotracker signals, indicative of lysosomal malfunction ( Fig. 3 ). Although spin homozygous flies underwent progressive neurodegeneration [4] , [8] , mosaic flies carrying spin mutant cells did not suffer from a similar symptom, presumably because nearby wild-type ( spin heterozygous) cells complemented, at least in part, functional deficits in spin mutant cells. We therefore consider that the behavioural phenotype observed in these mosaic flies is not an indirect consequence of global neurodegeneration. An alternative possibility is that not only ‘ionotropic’ (electrical activity) but also ‘metabotropic’ (molecular signalling) functions are important for these neurons to attain a high level of female sexual receptivity, and the Spin protein is the critical component in the latter process. Indeed, Spin is an important signalling molecule that mediates cell death [4] , [8] and lysosome reformation associated with mTOR activation following starvation [19] , [20] . Spin is also suggested to be an efflux permease that mediates release of lysosomal digests into cytosol [19] . The mTOR signalling pathway composes the core system for the homoeostasis of nutritional states [31] , [32] . Mating induces drastic changes in nutritional demands in females as they begin massive production of eggs to oviposit after copulation. In fact, females develop a preference for protein-rich diets after mating, and this change in food preference appears to be mediated by mTOR signalling [32] , which is, in part, stimulated by the neural action of the sex peptide transferred from a male during copulation [31] , [33] . An attractive hypothesis is that the food preference and sexual receptivity in females are both regulated by mTOR signalling, in which Spin is involved. Our study has identified two neuronal groups critically involved in the regulation of sexual receptivity, and this opens the way to elucidation of the sophisticated decision-making circuitry for adaptive changes in female behaviour at the single-cell level. Flies Flies were raised on a cornmeal-agar-yeast medium at 25 °C. The variants we used are described in the FlyBase database ( http://flybase.org/ ). Wild-type Canton-S flies were used as the control. spin P1 and spin P2 are strains carrying a P -element insertion at the spin locus, and were described in Nakano et al [4] . All RNAi strains were purchased from the Vienna Drosophila RNAi Center. elav c155 , an enhancer-trap GAL4 driver, was used to induce UAS-spin + type I , UAS-spinRNAi or UAS-TOR.TED expression in all neurons and repo-GAL4 in most of glia. To enhance the knockdown effect, UAS-dicer-2 was introduced into the flies. Chat-GAL80 ( [34] ) was used to inhibit the GAL4 function in cholinergic neurons. Behavioural assays The animals were raised at either 25 or 29 °C by the time of mating behaviour assays, which were conducted at 25 °C. To observe mating behaviour, virgin females were collected at eclosion and placed individually in food vials for 4–7 days. Each female fly was transferred to a round mating chamber (8 mm in diameter; 3 mm in height) with a wild-type virgin male. The behaviour of the fly pair was recorded using a video recorder. To estimate the level of female sexual receptivity, the cumulative number of copulating pairs in a 1-h observation period was counted and the average time to copulation was compared among the fly groups subjected to different types of manipulation or different genotypes. MARCM analysis of female sexual behaviour Somatic clones were produced using the MARCM method as described previously [5] . The flies used for MARCM analysis were obtained by crossing females of y hs-flp; FRTG13 tub-Gal80 and males of w; FRTG13 UAS-mCD8::GFP spin P2 /CyO; spin-GAL4. Embryos were collected within 24 h of egg laying and heat-shocked at 37 °C for 180 min. The mating behaviour assays for the mosaic flies were essentially identical to those described above, except that the single females were tested twice with a different male to minimize the inclusion of false-negative events in which the female fortuitously failed to copulate (irrespective of the spin genotype) in the first test. Histology Fixation and immunohistochemical staining were carried out as described previously [35] using the following antibodies and dilutions: rabbit polyclonal anti-GFP (1:1,000; Molecular Probes, Eugene, OR), rat monoclonal anti-Elav (1:100; Developmental Studies Hybridoma Bank, Iowa city, IA), mouse monoclonal anti-Repo (1:50; Developmental Studies Hybridoma Bank), mouse monoclonal nc82 (1:20; Developmental Studies Hybridoma Bank), Alexa488-conjugated goat anti-rabbit IgG (1:200; Invitrogen, Carlsbad, CA) and Alexa546-conjugated goat anti-mouse IgG (1:200; Invitrogen). To label lysosomes, brains were stained with 100 nM Lysotracker Red DND-99 (Molecular Probes) for 30 min without fixation. Stacks of optical sections at 1 or 2 μm were obtained with an LSM 510 META confocal microscope (Carl Zeiss, Oberkochen, Germany) and were processed with ImageJ software (ver. 1.40g). How to cite this article: Sakurai, A. et al. Select interneuron clusters determine female sexual receptivity in Drosophila . Nat. Commun. 4:1825 doi: 10.1038/ncomms2837 (2013).